Phase evolution for conversion reaction electrodes in lithium-ion batteries The performance of battery materials is largely governed by structural and chemical evolutions during electrochemical reactions. Therefore, resolving spatially dependent reaction pathways could enlighten mechanistic understanding, and enable rational design for rechargeable battery materials. Here, we present a phase evolution panorama via spectroscopic and three-dimensional imaging at multiple states of charge for an anode material (that is, nickel oxide nanosheets) in lithium-ion batteries. We reconstruct the three-dimensional lithiation/delithiation fronts and find that, in a fully electrolyte immersion environment, phase conversion can nucleate from spatially distant locations on the same slab of material. In addition, the architecture of a lithiated nickel oxide is a bent porous metallic framework. Furthermore, anode–electrolyte interphase is found to be dynamically evolving upon charging and discharging. The present study has implications for resolving the inhomogeneity of the general electrochemically driven phase transition (for example, intercalation reactions) and for the origin of inhomogeneous charge distribution in large-format battery electrodes. Phase conversions are ubiquitous and fundamentally important in many aspects of materials science research including colloidal synthesis [1] and lithium chemistry [2] , [3] . The response of a material to phase conversions on the nanoscale can directly dictate the performance of various energy materials in electrochemical reactions, such as fuel cell nanocatalysts [4] , [5] and battery electrodes [2] , [3] , [6] , [7] , [8] , [9] , [10] , [11] , [12] , [13] . Specifically, phase conversion reactions have provided a rich playground for lithium-ion battery technologies with potential to improve specific/rate capacity and achieve high resistance to lithium metal plating [14] , [15] , [16] , [17] , [18] , [19] . Among the many potential candidates, transition metal oxides have received broad interests as lithium-ion battery anode materials [20] , [21] , [22] , [23] , [24] , [25] , [26] , [27] . Although electrochemistry and synthesis of transition metal oxides have been well studied [18] , [19] , the spatially resolved phase conversion pathways (for example, nucleation, charge distribution and anode–electrolyte interface (AEI) formation) remain elusive. To understand these nanoscale pathways could impart knowledge not only to unravel the underlying mechanism/challenges of conversion reactions [28] but also to reveal the origin of inhomogeneous charge distribution in large-format battery electrodes [10] , [29] , [30] . In recent years, in situ transmission electron microscopy (TEM) studies have been performed to investigate the electrochemically driven phase conversions in lithium-ion batteries. However, most of these studies primarily focused on non-volatile environments and lacked information on interfaces between commercially used organic liquid electrolytes and battery electrodes [8] , [11] . Furthermore, due to limitations of TEM sample geometry in these studies, electrode–electrolyte interfaces were simplified as a point/line contact and thus failed to represent the electrode materials’ three-dimensional (3D) immersion in electrolyte that occurs in practical battery cells. Other groups have attempted quasi in situ observation of energy materials supported on TEM grids in liquid electrochemical cells [31] . However, due to the limited loading allowed on a TEM grid, an accurate and reproducible charging/discharging rate (C-rate) control is difficult to achieve but is essential for lithium-ion battery systems. Here, we report a direct visualization of phase conversion in a high performance anode material in a coin cell configuration. In the coin cell, we pressed a holey carbon supported TEM grid, which was loaded with a small amount of the anode material, against the bulk anode to ensure that the materials on the grid are submerged in the same electrolyte environment as the bulk anode ( Fig. 1 ). This configuration allows us to accurately control the C-rate for cycling; in addition, the TEM grid can be dissembled from the cell to facilitate TEM imaging and spectroscopy. This grid-in-a-coin cell methodology has enabled direct probing of the 3D morphology and charge state distribution of the anode material and evolution of AEI at different stages of electrochemical cycling with atomic-scale TEM imaging, electron tomography, electron energy loss spectroscopic mapping as well as ensemble-averaged synchrotron X-ray spectroscopy. 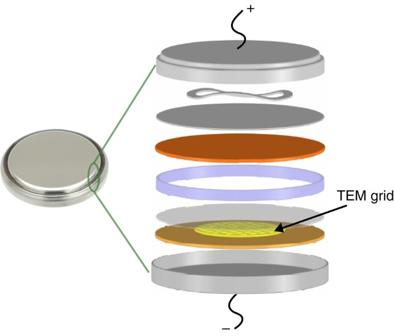Figure 1: Schematic illustration of a coin cell design loaded with a TEM grid. In the coin cell, a holey carbon supported TEM grid, which was loaded with a small amount of the anode material, was pressed against the bulk anode to ensure the materials on the grid are submerged in the same electrolyte environment as the bulk anode. From top to bottom: anode cap, spring, spacer, lithium anode, gasket, separator, TEM grid loaded with NiO nanosheets, working electrode and cathode cap. A NiO-based working electrode is considered as a ‘cathode’ in this half-cell configuration but as an ‘anode’ in the full-cell configuration. Therefore, a NiO-based working electrode is identified as an ‘anode’ in this paper. Figure 1: Schematic illustration of a coin cell design loaded with a TEM grid. In the coin cell, a holey carbon supported TEM grid, which was loaded with a small amount of the anode material, was pressed against the bulk anode to ensure the materials on the grid are submerged in the same electrolyte environment as the bulk anode. From top to bottom: anode cap, spring, spacer, lithium anode, gasket, separator, TEM grid loaded with NiO nanosheets, working electrode and cathode cap. A NiO-based working electrode is considered as a ‘cathode’ in this half-cell configuration but as an ‘anode’ in the full-cell configuration. Therefore, a NiO-based working electrode is identified as an ‘anode’ in this paper. Full size image Our charge mapping and 3D reconstructions of the electrochemically cycled materials reveal that during both lithiation and delithiation, phase conversions can initiate and propagate from spatially distant locations on the same slab of anode material. This suggests a heterogeneous phase conversion mechanism, analogous to heterogeneous nucleation in crystal growth, can be dominant and fundamentally important in the conversion reaction. The present study captures previously unexpected heterogeneous nucleation characteristics in electrochemically driven phase conversions in metal oxides, providing insights into designing practically viable conversion reaction electrodes in general. Morphology and electronic structure of NiO nanosheets Owing to its high theoretical capacity, NiO and its nanocomposites have been extensively studied as potential anodes for high-capacity lithium-ion batteries [18] , [19] . Here, structurally well-defined NiO material was prepared using a solvothermal method aided with a pseudo-supercritical drying technique [32] . The as-prepared NiO exhibits a sheet-like structure with hexagonal holes ( Fig. 2a,b ) and a thickness of 24±8 nm ( Supplementary Fig. 1 ). The atomic resolution annular dark-field scanning TEM (ADF-STEM) image reveals that nickel ions are packed into a hexagonal arrangement with the zone axis aligned perpendicular to the nanosheet ( Fig. 2c ) indicating that the surface primarily consists of rock salt (111) facets. The formal oxidation state of nickel is 2+ in NiO nanosheets as determined by soft X-ray absorption spectroscopy (XAS) and spatially resolved electron energy loss spectroscopy (EELS), both of which correspond to the dipole allowed transitions from Ni 2p 6 3d 8 to Ni 2p 5 3d 9 states, including Ni 2p 3/2 and Ni 2p 1/2 spin-orbit final states [33] , [34] ( Fig. 2d,e ). The pre-edge feature in the O K-edge corresponds to the p-character of the Ni3d-O2p hybridized states in the NiO 6 octahedral unit [35] . The O K-edge feature associated with Ni3d-O2p hybridization states in the pristine NiO nanosheet is equivalently observed using XAS and EELS ( Fig. 2d,e ). The consistency between XAS and EELS suggests the homogeneity of the pristine material and demonstrates the capability of performing correlated studies for efficient phase identification and charge mapping. 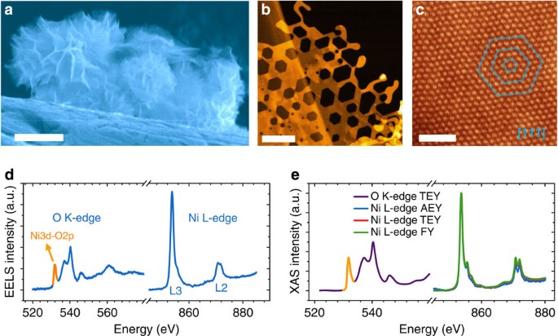Figure 2: Pristine NiO nanosheets. (a) SEM image of NiO nanosheet bundles supported on a stainless steel substrate. (b) ADF-STEM overview image of an individual NiO nanosheet. (c) ADF-STEM image of a NiO nanosheet along the [111] zone axis. The hexagons are drawn for the visual enhancement of the hexagonal arrangement of nickel ion columns. (d) EELS O K-edge and Ni L-edge spectra for a NiO nanosheet (~0.8 eV energy resolution). (e) XAS O K-edge and Ni L-edge spectra for a pristine NiO electrode, where the XAS O K-edge spectrum was collected using TEY mode and XAS Ni L-edge spectra were collected using AEY, TEY and FY modes. XAS Ni L-edge spectra show the bulk and surface consistency of the pristine NiO electrode. The scale bars are 5 μm, 100 nm and 1 nm in (a), (b) and (c), respectively. Figure 2: Pristine NiO nanosheets. ( a ) SEM image of NiO nanosheet bundles supported on a stainless steel substrate. ( b ) ADF-STEM overview image of an individual NiO nanosheet. ( c ) ADF-STEM image of a NiO nanosheet along the [111] zone axis. The hexagons are drawn for the visual enhancement of the hexagonal arrangement of nickel ion columns. ( d ) EELS O K-edge and Ni L-edge spectra for a NiO nanosheet (~0.8 eV energy resolution). ( e ) XAS O K-edge and Ni L-edge spectra for a pristine NiO electrode, where the XAS O K-edge spectrum was collected using TEY mode and XAS Ni L-edge spectra were collected using AEY, TEY and FY modes. XAS Ni L-edge spectra show the bulk and surface consistency of the pristine NiO electrode. The scale bars are 5 μm, 100 nm and 1 nm in ( a ), ( b ) and ( c ), respectively. Full size image Electrochemical performance of NiO nanosheets Charge–discharge voltage profile shows distinct phase conversion plateaus for the NiO/Ni redox couple ( Fig. 3a ). The NiO reduction potentials are 0.6 V and 1.0–1.5 V for the first cycle and subsequent cycles, respectively. The charge–discharge redox behaviour remained intact when a TEM grid was included in the coin cell ( Supplementary Fig. 2 ). 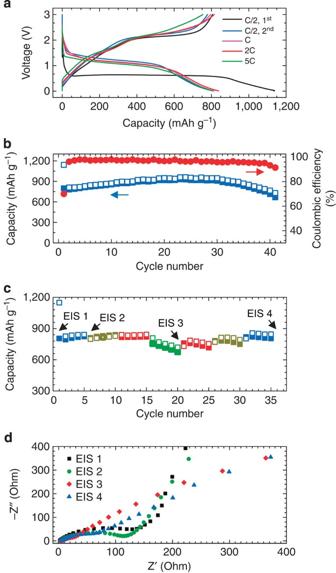Figure 3: Battery cycling performance of NiO nanosheets. (a) Charge–discharge voltage profiles at different C rates. (b) Capacity retention (left y-axis) and coulombic efficiency (right y-axis) at C/2 rate. (c) Rate capability: C/2 (blue), C (yellow), 2C (red) and 5C (green). (d) Electrochemical impedance Nyquist plots after charge–discharge cycles and the corresponding EIS collection points are indicated in (c). The charge capacity and discharge capacity are indicated, respectively, by solid and open cubes in (b) and (c). Supplementary Figure 3 shows the cyclic voltammetry for the first two cycles, where the voltage ranges corresponding to the NiO reduction potentials are identified. At C/2, the first discharge and charge capacities are 1,138 mAh g −1 and 808 mA g −1 , respectively. The first cycle coulombic inefficiency is attributed to the incomplete decomposition of AEI and other factors including kinetic limitations in the charging process [26] . The charge–discharge voltage hysteresis showed negligible change at different C rates ( Fig. 3a ), which suggests that the reaction pathway remained intact [18] . Coulombic efficiency is improved to 98% for the second cycle at C/2 and shows little degradation with extended charge–discharge cycles ( Fig. 3b ). Specific charge capacity reaches a peak of 928 mAh g −1 and remains remarkably high (675 mAh g −1 ) after 40 cycles ( Fig. 3b ). The higher capacity relative to the theoretical capacity (718 mAh g −1 ) suggests that interfacial charge storage and/or reversible side reactions play roles in the extra capacity [22] , [36] . The reversible side reactions probably include but are not limited to lithium storage in carbon black [37] and CuO [38] at the surface of the Cu current collector, and reversible conversion of LiOH to Li 2 O and LiH [39] . An extraordinary high-rate capability is demonstrated in Fig. 3c in which the cell retains a specific capacity of 755 mAh g −1 at 5C and is fully recovered at C/2 after a series of high-rate charge–discharge cycles. Impedance Nyquist plots were collected after high-rate cycling and are shown in Fig. 3d . The Nyquist spectra are composed of semicircles at high frequency and Warburg tails at low frequency. The semicircles include both charge transfer resistance and thin film resistance. Detailed analysis of the semicircles is provided in Supplementary Fig. 4 and Supplementary Table 1 . Briefly, the thin film resistance was gradually increased after charge–discharge cycles due to the AEI formation. However, the charge transfer resistance underwent significant reduction after charge–discharge cycles, especially after high-rate cycling ( Fig. 3d , Supplementary Fig. 4 and Supplementary Table 1 ), which suggests that the superior rate capability is probably attributed to the improved charge transfer. Overall, the electrochemical performance of NiO nanosheets is superior to the reported NiO anode materials in the literature [25] , [40] , which renders NiO nanosheets an excellent candidate to study phase change in conversion reactions. Furthermore, NiO is a member of the conversion reaction family and its behaviour is expected to be transferrable to other high performance 3d transition metal oxide anodes such as Fe 2 O 3 , CoO and MnO 2 . Figure 3: Battery cycling performance of NiO nanosheets. ( a ) Charge–discharge voltage profiles at different C rates. ( b ) Capacity retention (left y-axis) and coulombic efficiency (right y-axis) at C/2 rate. ( c ) Rate capability: C/2 (blue), C (yellow), 2C (red) and 5C (green). ( d ) Electrochemical impedance Nyquist plots after charge–discharge cycles and the corresponding EIS collection points are indicated in ( c ). The charge capacity and discharge capacity are indicated, respectively, by solid and open cubes in ( b ) and ( c ). Full size image Surface chemistry and phase conversion in NiO nanosheets To begin with, we achieved ensemble-averaged characteristics for composite electrodes under various states of charge (SOC). The intensity of XAS in the Auger electron yield (AEY) mode is sensitive to the overlayer thickness ( d ) at the surface of a material due to the limited mean free path of Auger electrons in the overlayer. Under identical Auger electron signal collection configurations, the AEY intensity is empirically in an exponential relationship with (− d ). Therefore, any chemical build-up at the surface of NiO nanosheets is evidenced by the decreased intensity of XAS in the AEY mode. Here, we observe that the Ni L-edge AEY intensity is dynamically altered depending on the SOC. As shown in Fig. 4a , the AEY signal was completely quenched in the fully discharged electrode and partially recovered in the charged state. This observation suggests that electrochemical processes govern the thickness of the surface overlayer, that is, the surface overlayer was developed and decomposed during discharging and charging, respectively. The normalized Ni L-edge spectra ( Supplementary Fig. 5 ) clearly show the changes of nickel oxidation states corresponding to the phase conversion plateaus in the charge–discharge voltage profiles ( Fig. 3a ). A comparison of XAS O K-edge spectra for the pristine and cycled electrodes provides direct evidence for chemical evolution in a large scale. As shown in Fig. 4b , the characteristic O K-edge peak associated with the Ni3d-O2p hybridization state is significantly degraded. In contrast, the intensity related to π*(C=O) [41] experiences dramatic enhancement in the cycled electrode (red spectrum in Fig. 4b ). The π*(C=O) is likely attributed to carbonate groups at the surface of nanosheets (see discussion below). The overlayer on nanosheets was visually confirmed by STEM imaging, and it is found that the overlayer occupies the surfaces of both NiO and Ni patches. A vast number of EELS spectra were acquired in the low-dose mode for the overlayer (that is, AEI) and the representative spectra are shown in Fig. 4d . The existence of carbonate groups is further confirmed with EELS C K-edge, where the sharp peak at 292.5 eV and the broad peak centred at 302.8 eV are attributed to the unoccupied π* and σ* antibonding molecular orbitals of CO 3 2− clusters [42] . (Careful alignment of EELS energy axis was performed by cross aligning the C K-edge of the nearby amorphous carbon with the standard spectrum.) The major feature of EELS O K-edge is in accordance with that observed in XAS O K-edge. Furthermore, the EELS Li K edge spectrum is in agreement with that reported for Li 2 CO 3 (ref. 43 ). In addition, localized Li 2 CO 3 nanocrystals were observed using high-resolution TEM imaging and fast Fourier transform ( Supplementary Fig. 6 ). Finally, one may conclude that the AEI likely consists of Li 2 CO 3 domains in a complex amorphous organic matrix, which is similar to those reported for graphite anode materials [44] , [45] , [46] , [47] . 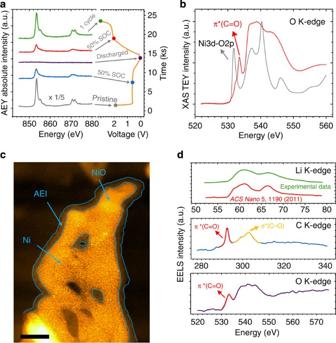Figure 4: Chemical evolution at the surface of NiO nanosheets. (a) XAS/AEY spectra for electrodes at different SOC, and the voltage-time profile is provided in parallel to indicate the states where data collection was accomplished. XAS/AEY is a surface detection mode and the Ni L-edge signal disappears at the fully discharged state due to a thick coating of AEI on the surface. (b) XAS/TEY O K-edge spectra for electrodes in the pristine state (grey) and in the 50% SOC (red), and the assignment of peaks is indicated in the figure. (c) STEM image of a NiO nanosheet during a discharging process, and NiO, Ni and AEI are indicated with arrows in the image. The scale bar is 50 nm. (d) EELS Li K-edge, C K-edge and O K-edge spectra for the AEI layer, and the assignment of peaks is indicated in the figure. A reference Li K-edge spectrum of Li2CO3(ref.43) is provided in the figure. Figure 4: Chemical evolution at the surface of NiO nanosheets. ( a ) XAS/AEY spectra for electrodes at different SOC, and the voltage-time profile is provided in parallel to indicate the states where data collection was accomplished. XAS/AEY is a surface detection mode and the Ni L-edge signal disappears at the fully discharged state due to a thick coating of AEI on the surface. ( b ) XAS/TEY O K-edge spectra for electrodes in the pristine state (grey) and in the 50% SOC (red), and the assignment of peaks is indicated in the figure. ( c ) STEM image of a NiO nanosheet during a discharging process, and NiO, Ni and AEI are indicated with arrows in the image. The scale bar is 50 nm. ( d ) EELS Li K-edge, C K-edge and O K-edge spectra for the AEI layer, and the assignment of peaks is indicated in the figure. A reference Li K-edge spectrum of Li 2 CO 3 (ref. 43 ) is provided in the figure. Full size image Next, phase conversion process was studied and previously unknown characteristics were revealed for conversion reactions. 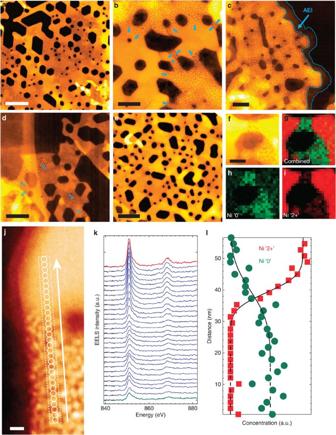Figure 5: STEM imaging and charge mapping. (a) Pristine NiO nanosheet. (b) NiO nanosheet with a 50% SOC (discharging). (c) NiO nanosheet with a fully discharged state. (d) NiO nanosheet with a 50% SOC (charging). (e) NiO nanosheet with a full cycle. (f–i) Charge mapping for a localized region with a 50% SOC, where (f), (g), (h) and (i) are STEM image, combined mapping profile, Ni ‘0’ mapping (green) and Ni ‘2+’ mapping (red), respectively. (j–l) EELS line profile, where (j), (k) and (l) are STEM image, EELS spectra and Ni ‘0’/Ni ‘2+’ concentration profiles, respectively. The arrows in (b) and (d) indicate the propagation direction of NiO-to-Ni and Ni-to-NiO conversions, respectively. The scale bars are 100 nm, 50 nm, 50 nm, 50 nm, 100 nm, 20 nm and 5 nm in (a), (b), (c), (d), (e), (f) and (j), respectively. Figure 5a–e show the representative STEM images for NiO nanosheets with various SOC. Electrochemically driven phase conversion has been interpreted as a progressive nucleation/propagation from the surface of a particle until the particle is fully converted, that is, core/shell model or homogeneous phase conversion [48] . In reality, conditions for homogenous phase conversion are hardly satisfied on the nanoscale, and any fluctuations on the electrolyte exposure, electrical contact or crystal defects will foster heterogeneous phase conversion. Our observation reveals that heterogeneous phase conversion can be dominant even in ultrathin nanosheets. Figure 5b,d demonstrate heterogeneous phase conversion phenomena during lithiation and delithiation processes, respectively. During lithiation, nanoscale nickel networks preferentially nucleate in a number of spatially distant locations on a single NiO nanosheet and then propagate into the vicinity until the propagation fronts meet, as indicated by the arrows in Fig. 5b . The opposite reaction, NiO formation, exhibits nearly identical heterogeneous characteristics, as shown in Fig. 5d . Supplementary Figure 7 provides more S/TEM images for the heterogeneous phase conversion phenomena. 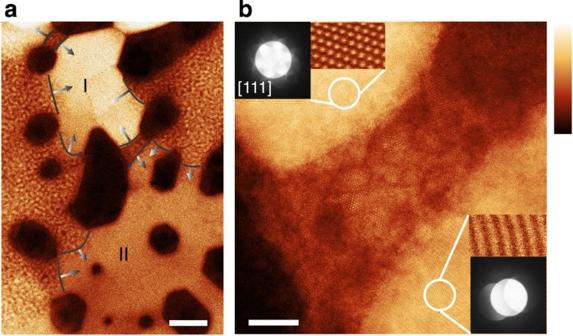Figure 7: Propagation of heterogeneous nucleation at grain boundaries. (a) Low-magnification high-angle ADF-STEM (HAADF-STEM) image showing heterogeneous nucleation with multiple nucleation fronts indicated by bending contours and arrows. (b) Atomic resolution HAADF-STEM image for a selected phase conversion scene, where the insets show atomic arrangements and convergent beam electron diffraction patterns for NiO patch I and NiO patch II in (a). The scale bars are 30 nm and 5 nm in (a) and (b), respectively. After a full cycle, the majority of NiO nanosheets were retained in the crystalline structure, as shown in Fig. 5e . The lattice resolution image of the delithiated NiO material and the bending contours in the low-magnification TEM image ( Supplementary Fig. 8 ) clearly demonstrate that the cycled NiO remains crystalline with a crystalline domain size of ~100 nm. Charge distribution mapping was performed on a region with heterogeneous phase conversion using Ni L-edge EELS spectroscopy, as shown in Fig. 5f–i . The mapping provides a direct visualization for the lithiation process. The area coloured in green represents the NiO that has already been converted to Ni metal, while no phase conversion has occurred in the area coloured in red. EELS line scans were performed at the vicinity of a phase propagation front, as shown in Fig. 5j . Scanning from the pure Ni region to the pure NiO region ( Fig. 5j ), we observed a gradual evolution in the shapes and intensities of Ni L 2,3 near-edge fine structures due to the variation of nickel oxidation states ( Fig. 5k ). The spectra with mixed nickel oxidation states could be decomposed using a linear combination of Ni 0 and Ni 2+ fingerprints, Ni 0 and Ni 2+ profiles are plotted as a function of the relative position along the scanning line ( Fig. 5j ). In general, Ni 0 and Ni 2+ profiles exhibit opposite trends along the scanning direction. A mixed-state region was observed at the boundary between the pure Ni 0 region and the pure Ni 2+ region ( Fig. 5l ). This asymmetric distribution of nickel valence states suggests a unidirectional propagation of the phase conversion front, which is a characteristic of heterogeneous phase conversion. Figure 5: STEM imaging and charge mapping. ( a ) Pristine NiO nanosheet. ( b ) NiO nanosheet with a 50% SOC (discharging). ( c ) NiO nanosheet with a fully discharged state. ( d ) NiO nanosheet with a 50% SOC (charging). ( e ) NiO nanosheet with a full cycle. ( f – i ) Charge mapping for a localized region with a 50% SOC, where ( f ), ( g ), ( h ) and ( i ) are STEM image, combined mapping profile, Ni ‘0’ mapping (green) and Ni ‘2 + ’ mapping (red), respectively. ( j – l ) EELS line profile, where ( j ), ( k ) and ( l ) are STEM image, EELS spectra and Ni ‘0’/Ni ‘2+’ concentration profiles, respectively. The arrows in ( b ) and ( d ) indicate the propagation direction of NiO-to-Ni and Ni-to-NiO conversions, respectively. The scale bars are 100 nm, 50 nm, 50 nm, 50 nm, 100 nm, 20 nm and 5 nm in ( a ), ( b ), ( c ), ( d ), ( e ), ( f ) and ( j ), respectively. 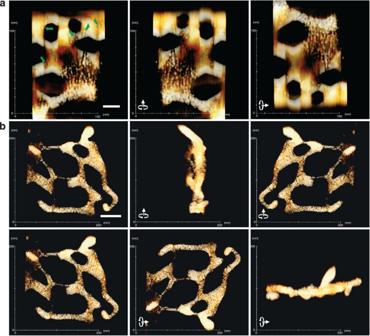Full size image The visualization of a heterogeneous phase conversion was achieved by reconstructing the 3D internal nanostructures for a nanosheet with 50% SOC (during the charging process) by ADF-STEM tomography. Figure 6: 3D STEM tomography. (a) A reconstructed NiO nanosheet with 50% SOC during charging process, and the green arrows exemplify the Ni nanoparticles that are imbedded in the NiO matrix as a result of heterogeneous nucleation. (b) A reconstructed NiO nanosheet in the fully discharged state. The electrochemically reduced Ni forms a bent porous metallic framework. The rotation operations are indicated in the figures. SeeSupplementary Informationfor complete movies (Movies 1 and 4). The scale bars are 20 nm and 50 nm in (a) and (b), respectively. Figure 6a shows the snapshots for the reconstructed tomography on different orientations, and the associated full-view movie is provided in Supplementary Movie 1 . Nickel nanoparticles are discernible in the NiO matrix close to the propagation fronts that are indicated by the green arrows in Fig. 6a . These imbedded nickel nanoparticles would otherwise be ignored in projection images but validate the mixed nickel oxidation state at the boundary between the pure Ni 0 region and the pure Ni 2+ region ( Fig. 5l ). Furthermore, we noticed the morphology of the Ni 0 region was different from the conventional understanding [20] , [24] , [49] , [50] , [51] . With projection images, it is possible to incorrectly perceive that individual discrete Ni nanoparticles are imbedded in the complex compounds containing Li, O and C [20] , [24] , [49] , [50] . However, projection images could be misleading in terms of distinguishing chemically interconnected nanoparticles from physically overlapped nanoparticles. True morphology can only be visualized by 3D tomography. In the lithiated region of Fig. 6a , nickel nanoparticles are interconnected into a porous network and exhibit greatly distinct characteristics in contrast to the widely accepted model of discrete spherical metal nanoparticles [20] , [24] , [49] , [50] . The interconnected nickel networks are further supported by the high-magnification reconstructed tomography of the lithiated region, as shown in Supplementary Movie 2 . The heterogeneous nucleation phenomenon is also dominant during the discharging process, and the reconstructed images are shown in Supplementary Fig. 9 and Supplementary Movie 3 . The porous metallic structure is completely retained towards the end of a discharging process, as shown in Fig. 6b . Supplementary Movie 4 illustrates the full-view panorama for the interconnecting framework. Finally, the benefit of the 3D metallic framework not only lies in the improved electron transfer but also the structural integrity (that is, inhibit pulverization) of NiO nanosheets thus allowing for durable high-rate cycling. This is direct evidence of a nanoporous metallic framework in conversion reactions. The result suggests that enhanced durability could be realized for conversion reaction electrodes if appropriate cycling conditions are applied to exclusively yield nanoporous frameworks. It is noted that pore size in the framework is much smaller than electrochemically dealloyed metallic porous structures in the literature [52] , which enables potential applications of the present porous frameworks in catalysis and sensing. Another unexpected phenomenon is the bending of nanosheets after a complete lithiation step ( Fig. 6b and Supplementary Movie 4 ), which is rarely observed after a complete delithiation step. We infer that the bending phenomenon is largely attributed to the electrochemically induced plastic deformation of the metallic porous framework. Presumably, the energy associated with the plastically deformed bending originates from the electrical energy supplied by the external circuit during the discharging process. Therefore, the reversibility of such bending under extended charge–discharge cycles should impose effects on the efficiency of battery cycling. Figure 6: 3D STEM tomography. ( a ) A reconstructed NiO nanosheet with 50% SOC during charging process, and the green arrows exemplify the Ni nanoparticles that are imbedded in the NiO matrix as a result of heterogeneous nucleation. ( b ) A reconstructed NiO nanosheet in the fully discharged state. The electrochemically reduced Ni forms a bent porous metallic framework. The rotation operations are indicated in the figures. See Supplementary Information for complete movies (Movies 1 and 4). The scale bars are 20 nm and 50 nm in ( a ) and ( b ), respectively. Full size image Mechanism of heterogeneous nucleation in NiO nanosheets The origin of heterogeneous phase conversion could be attributed to inhomogeneous electrolyte exposure, electrical contact and/or intrinsic crystal defects, such as grain boundaries. It is unlikely the origin of heterogeneous nucleation at the atomic scale will be elucidated using X-ray based imaging techniques [48] , [53] . Specifically, we observed that Ni nucleation preferentially emerges at grain boundaries, as shown in Fig. 7a . The orientations of the two patches of NiO are not registered, as demonstrated by the channelling contrast ( Fig. 7a ), convergent beam electron diffraction patterns (insets of Fig. 7b ), and atomically resolved HAADF-STEM images (insets of Fig. 7b ), indicating that there was likely a grain boundary present between the two patches before lithiation. This observation suggests that electrochemically driven phase conversion follows the fundamental rules of phase transformation in solids that nucleation activation energy is lower at grain boundaries due to the extra energy associated with lattice distortion and dislocations [54] . In addition, the loosely packed lattices along grain boundaries create a rapid diffusion channel for lithium ions therefore enabling the nucleation of nickel metal nanoparticles. Figure 7: Propagation of heterogeneous nucleation at grain boundaries. ( a ) Low-magnification high-angle ADF-STEM (HAADF-STEM) image showing heterogeneous nucleation with multiple nucleation fronts indicated by bending contours and arrows. ( b ) Atomic resolution HAADF-STEM image for a selected phase conversion scene, where the insets show atomic arrangements and convergent beam electron diffraction patterns for NiO patch I and NiO patch II in ( a ). The scale bars are 30 nm and 5 nm in ( a ) and ( b ), respectively. Full size image The elucidation of electrochemically driven phase conversion is fundamentally significant to interpret electrode behaviours for rechargeable batteries. On account of the unique two-dimensional morphology of NiO nanosheets, we were able to resolve phase conversion characteristics in a battery electrode using both spatially resolved and ensemble-averaged diagnostic tools. Our finding probes the nanoscale phase conversion and chemical evolution phenomena that are directly associated with the battery performance in practice. Firstly, the chemical environment of AEI at the surface of NiO nanosheets is determined to be Li 2 CO 3 nanoscale domains imbedded in an amorphous organic matrix and its thickness exhibits dependence on the SOC. The chemical environment of AEI on NiO nanosheets is similar to that at the surface of graphite anode materials [44] , [46] , [47] . Therefore, these observations represent a step towards leveraging AEI on transition metal oxide materials with the conventional concept of solid–electrolyte interphase on graphite materials [28] , [45] . Secondly, the electrochemically produced nickel nanoparticles are constructed into a bent nanoporous metallic framework that inhibits pulverization and maintains the integrity of NiO nanosheets to allow extended charge–discharge cycles. This result resolves the previous misconception about the morphology of transition metal nanostructures that were exclusively identified as discrete nanoparticles [20] , [24] , [49] , [50] , amorphous domains [51] or localized interconnected nanoparticles [7] . Furthermore, the nanoporous framework creates an electron diffusion network to enable high-rate capability for conversion reactions [55] . Thirdly, heterogeneous phase conversion was found to prevail in conversion reactions, which is likely caused in part by the preferential nucleation at grain boundaries. Presumably, the particles with different densities of grain boundaries undergo phase conversion at different rates resulting in inhomogeneous charge distribution in large-format batteries. Previous in situ TEM studies observed unidirectional phase propagation phenomena using a single point/line contact [8] . Our results show that the unidirectional phase propagation mechanism is still valid to some degree under more relevant battery conditions, for example, the present coin cell configuration. However, in particles with 3D electrolyte immersion and electrical contact, multiple propagation fronts proceed simultaneously in each individual nanosheet, and the phase propagation event is completed when the propagation fronts merge. This phenomenon has been overlooked in the imaging techniques that lack atomic resolution (for example, synchrotron X-ray imaging). Finally, the discrepancy between our study and a recently reported core-shell model [48] is attributed to the different spatial resolution achieved in these studies. The atomic-scale investigation in the present study enriches the mechanistic paradigm for phase conversion phenomena at a complementary length scale. In summary, on the basis of the high performance NiO nanosheets, the present study delivers completely new insights into phase conversion and chemical evolution of transition metal oxides in atomic scale and sheds light on the inhomogeneous charge distribution in large-format battery electrodes. Electrode preparation and battery testing The active material (NiO nanosheets) was synthesized using a solvothermal method aided with an alcohol pseudo-supercritical drying technique. Ni(NO 3 ) 2 ·6 H 2 O, urea and benzyl alcohol was added into 50 ml of methanol with a molar ratio of 2:1:4. The solution was stirred for 1 h and transferred to an autoclave (Parr Reactor, model #4520). The reaction mixture was purged with Ar for 1 min and then Ar was filled with a pressure of 9 bars before initiating the heating process. The mixture was heated to 265 °C and maintained for 1.5 h. Finally, the vapour inside was vented (that is, pseudo-supercritical drying process). A green powder was collected and was subsequently calcined at 500 °C for 6 h to yield NiO nanosheets. Composite electrodes were prepared with 80 wt% active material, 10 wt% polyvinylidene fluoride and 10 wt% acetylene carbon black in N -methyl-2-pyrrolidone and cast onto copper current collectors with loadings of 1–2 mg cm −2 . The packing density was calculated to be 0.7 g cm −3 using the areal loading divided by the cross-sectional thickness of the electrode ( Supplementary Fig. 10 ). 2032-type coin cells were assembled in an argon-filled glove box using the composite electrode as the positive electrode and Li metal as the negative electrode. A Celgard separator 2400 and 1 M LiPF 6 electrolyte solution in 1:1 w/w ethylene carbonate/diethyl carbonate were used to fabricate coin cells. Battery testing was performed on computer controlled VMP3 channels (BioLogic). 1C was defined as full discharging NiO in 1 h, which corresponds to a specific current density of 718 mA g −1 (NiO has a theoretical capacity of 718 mAh g −1 ). The charging current was set identical to that of the discharging in the present study. Electrochemical impedance spectra were collected after full cycles with a 10 mV AC signal ranging from 10 mHz to 100 kHz. Cyclic voltammetry was performed with a scan rate of 0.5 mV s −1 . To achieve real battery cycling and nanoscale visualization in an identical configuration, a TEM grid loaded with NiO nanosheets was pressed against the composite electrode ( Fig. 1 ). The TEM grid was carefully removed and rinsed with diethyl carbonate after the designated electrochemical cycling and allowed to dry for an extended period of time in the glove box. Composite electrodes on copper foils and TEM grids were transferred under Ar protection for ensemble-averaged and spatially resolved measurements, respectively. Synchrotron XAS High-throughput XAS measurements were performed on the 31-pole wiggler beamline 10-1 at Stanford Synchrotron Radiation Lightsource using a ring current of 350 mA and a 1,000 l mm −1 spherical grating monochromator with 20 μm entrance and exit slits, providing ~10 11 ph s −1 at 0.2 eV resolution in a 1 mm 2 beam spot. During the measurements, all samples were attached to an aluminium sample holder, and the surface was connected to the isolated holder using conductive carbon. Data were acquired in a single load at room temperature and under ultrahigh vacuum (10 −9 torr). For TEY, we collected the sample drain current, and a silicon diode (IRD AXUV-100) was used to collect the fluorescence yield positioned near the sample surface. AEY was collected with a Cylindrical Mirror Analyser using a pass energy of 200 eV and a kinetic energy window of 2 eV near the main Auger for oxygen and nickel, respectively. Contributions from visible light were carefully minimized before the acquisition, and all spectra were normalized by the current from freshly evaporated gold on a fine grid positioned upstream of the main chamber. Samples were prepared by loading battery electrodes onto a conductive carbon tape, which was mounted on an aluminium holder attached to the main chamber manipulator. Electron microscopy and spectroscopy 200 and 300 keV field-emission S/TEMs were used for ADF-STEM tomographic imaging. EELS data sets were acquired using a Gatan Tridiem spectrometer. Tilt series images were recorded from −70° to +70° with 1° intervals. Tomograms were reconstructed using the e − Tomo software suite written by Robert Hovden et al. (Cornell Muller group) and visualized by Avizo 6.3. How to cite this article: Lin, F. et al. Phase evolution for conversion reaction electrodes in lithium-ion batteries. Nat. Commun. 5:3358 doi: 10.1038/ncomms4358 (2014).